Cytokinin response factors regulatePIN-FORMEDauxin transporters Auxin and cytokinin are key endogenous regulators of plant development. Although cytokinin-mediated modulation of auxin distribution is a developmentally crucial hormonal interaction, its molecular basis is largely unknown. Here we show a direct regulatory link between cytokinin signalling and the auxin transport machinery uncovering a mechanistic framework for cytokinin-auxin cross-talk. We show that the CYTOKININ RESPONSE FACTORS (CRFs), transcription factors downstream of cytokinin perception, transcriptionally control genes encoding PIN-FORMED (PIN) auxin transporters at a specific PIN CYTOKININ RESPONSE ELEMENT ( PCRE ) domain. Removal of this cis -regulatory element effectively uncouples PIN transcription from the CRF-mediated cytokinin regulation and attenuates plant cytokinin sensitivity. We propose that CRFs represent a missing cross-talk component that fine-tunes auxin transport capacity downstream of cytokinin signalling to control plant development. The hormones auxin and cytokinin are essential to control plant growth and development including early embryogenesis [1] , [2] and postembryonic organogenic processes, such as root [3] , [4] , [5] and shoot [6] branching, phyllotaxis [7] , shoot [8] , [9] and root apical meristem activity [10] , [11] and vascular development [12] , [13] . The principal pathways that manage their metabolism, distribution, and perception and the backbone molecular components have been identified [14] , [15] , [16] , [17] . Importantly, a complex network of interactions and feedback circuits interconnects both pathways and determines the final outcome of the individual hormone actions. Well-established are the mutual regulation of metabolic [18] and signalling pathways [2] , [8] , as well as the cytokinin-mediated modulation of auxin transport [10] , [11] , [12] . Cytokinin has been shown to influence cell-to-cell auxin transport by modification of the expression of several auxin transport components and thus to modulate auxin distribution important for root development [10] , [11] , [19] , [20] . Through the cytokinin receptor ARABIDOPSIS HISTIDINE KINASE3 (AHK3) and the downstream signalling components ARABIDOPSIS RESPONSE REGULATOR (ARR1) and ARR12, cytokinin has been shown to activate SHY2/IAA3 (SHY2), a repressor of auxin signalling that negatively regulates the PIN auxin transporters [10] . However, thus far, the components of the transcriptional complex that directly control PIN transcription in response to cytokinin are unknown. Here we show that the cytokinin response factors (CRFs) [21] transcriptionally control PIN-FORMED ( PIN ) genes encoding auxin transporters at a specific PIN CYTOKININ RESPONSE ELEMENT ( PCRE ) domain. Removal of this cis -regulatory element effectively uncouples PIN transcription from the CRF-dependent regulation and attenuates plant cytokinin sensitivity. Accordingly, plants with modified CRF activity exhibit alterations in the expression of PIN genes and developmental defects mimicking phenotypes of auxin distribution mutants. We propose that the CRFs act as components of the transcriptional regulatory complex, which mediates transcriptional control downstream of cytokinin and fine-tunes PIN expression during plant growth and development. The PCRE element mediates cytokinin-sensitive PIN7 expression To explore the upstream pathway mediating cytokinin-dependent PIN transcription, we searched for regulatory elements by a promoter-deletion analysis of the PIN7 and PIN1 promoters ( Supplementary Fig. 1a ). Initially, we focused on PIN7 of which transcription has previously been shown to be activated by cytokinin [11] , [12] . We confirmed that the promoter (1,423 bp upstream of the translational start site) of PIN7 fused to the green fluorescent protein ( GFP ) reporter gene ( Supplementary Fig. 1a ) is activated by cytokinin and that this region is sufficient to mediate the hormonal response ( Fig. 1a ). The abrupt change in the cytokinin response as a consequence of a 200-bp element deletion between 1,423 and 1,223 bp upstream of the ATG start codon hinted at the presence of a cis -regulatory element required for the cytokinin-mediated transcriptional control of PIN7 ( Fig. 1b ). The role of this regulatory element, designated as PCRE7 , in cytokinin-sensitive expression was further tested with a PIN7–GFP translational construct driven by the truncated ΔPIN7 promoter. Quantification of the membrane PIN7–GFP signal demonstrated that the expression, when driven by the truncated promoter, was largely insensitive to cytokinin treatment in the cells of the central root cylinder ( Fig. 1c–e ), as well as in the initials of lateral root primordial (LRP) ( Supplementary Fig. 2a–e ). The ΔPIN7 promoter activity was significantly weakened in the root provasculature and columella cells when compared with the full PIN7 promoter, indicating the importance of this promoter element for the regulation of the PIN7 steady-state expression ( Fig. 1a,c compared with Fig. 1b,d and e ). Hence, the loss of cytokinin sensitivity as a consequence of the promoter truncation implies the presence of a specific cis -regulatory element on which the cytokinin-susceptible transcriptional complex might act to fine-tune PIN7 expression in response to cytokinin. While the reason for the change in steady-state expression levels remains to be determined, based on the overlap between PIN7 expression and that of the TCS::GFP cytokinin-reponsive reporter in procambial cells [12] , we propose that cytokinin might, through this regulatory element, participate not only in the response to exogenously applied cytokinin but also in the establishment and maintenance of proper basal levels of PIN7 expression. 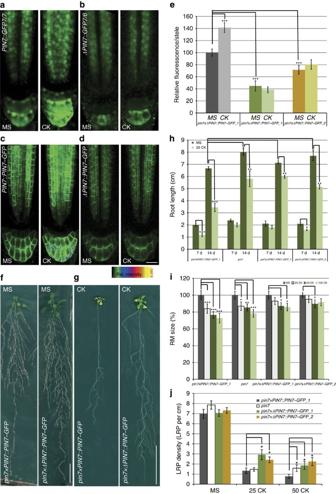Figure 1: Truncation ofPIN7promoter results in cytokinin-insensitivePIN7transcription. (a–e) Expression ofGFP(a,b) andPIN7–GFP(c,d) is upregulated in response to cytokinin when driven by the fullPIN7(a,c), but not the truncatedΔPIN7(b,d) promoter. Green: nuclear-localizedGFP(a,b); membrane-localizedPIN7–GFP(c,d). A semi-quantitative colour-coded heat map of the GFP fluorescence intensity is provided. Quantification ofPIN7–GFPin the provasculature of primary roots (e). Roots of 7-day-old seedlings (n=15) were treated with control Murashige and Skoog (MS) medium with or without 5 μM of the cytokinin (CK) N6-benzyladenine for 8 h. Student'st-test (***P<0.001,n=15). (f–j) Seedlings expressingΔPIN7::PIN7–GFPin thepin7background exhibit enhanced root growth (f,h) and reduced cytokinin sensitivity of primary root growth (f–h), root meristem (RM) size (i) and lateral root initiation (j). Seedlings were grown for 28 (f,g), 14 (h) and 7 days (d) (h–j) on MS medium with or without following cytokinins: 0.025 μM N6-benzyladenine (f–h); 0.025, 0.05 and 0.1 μM N6-benzyladenine (i); and 0.025 and 0.05 μM N6-benzyladenine (j). Student'st-test (*P<0.05;**P<0.01; ***P<0.001 (h,j); or *P<0.01;**P<0.001; ***P<0.0001 (i);n=10–15).ΔPIN7::PIN7–GFP_1andΔPIN7::PIN7–GFP_2represent two independent transgenic lines crossed into thepin7mutant background. Error bars represent s.e. Scale bars, 20 μm (a–d), 2 cm (f–g). Results were reproducible in three independent experiments. Figure 1: Truncation of PIN7 promoter results in cytokinin-insensitive PIN7 transcription. ( a – e ) Expression of GFP ( a , b ) and PIN7–GFP ( c , d ) is upregulated in response to cytokinin when driven by the full PIN7 ( a , c ), but not the truncated ΔPIN7 ( b , d ) promoter. Green: nuclear-localized GFP ( a , b ); membrane-localized PIN7–GFP ( c , d ). A semi-quantitative colour-coded heat map of the GFP fluorescence intensity is provided. Quantification of PIN7–GFP in the provasculature of primary roots ( e ). Roots of 7-day-old seedlings ( n =15) were treated with control Murashige and Skoog (MS) medium with or without 5 μM of the cytokinin (CK) N6-benzyladenine for 8 h. Student's t -test (*** P <0.001, n =15). ( f – j ) Seedlings expressing ΔPIN7::PIN7–GFP in the pin7 background exhibit enhanced root growth ( f , h ) and reduced cytokinin sensitivity of primary root growth ( f – h ), root meristem (RM) size ( i ) and lateral root initiation ( j ). Seedlings were grown for 28 ( f , g ), 14 ( h ) and 7 days (d) ( h – j ) on MS medium with or without following cytokinins: 0.025 μM N6-benzyladenine ( f – h ); 0.025, 0.05 and 0.1 μM N6-benzyladenine ( i ); and 0.025 and 0.05 μM N6-benzyladenine ( j ). Student's t -test (* P <0.05;** P <0.01; *** P <0.001 ( h , j ); or * P <0.01;** P <0.001; *** P <0.0001 ( i ); n =10–15). ΔPIN7::PIN7–GFP_1 and ΔPIN7::PIN7–GFP_2 represent two independent transgenic lines crossed into the pin7 mutant background. Error bars represent s.e. Scale bars, 20 μm ( a – d ), 2 cm ( f – g ). Results were reproducible in three independent experiments. Full size image Truncation of the PIN7 promoter disrupts plant growth Cytokinin-regulated plant growth and development has been proposed to be partly mediated by cytokinin-controlled PIN expression [10] , [11] . To dissect the developmental role of cytokinin-regulated PIN expression, plants expressing PIN7–GFP under the control of the truncated cytokinin-insensitive ΔPIN7 promoter or the wild-type PIN7 promoter were crossed with the pin7 mutant background and their seedlings were thoroughly inspected. Root growth analyses revealed that in young seedlings (7-day-old), growth of roots expressing either PIN7::PIN7–GFP/pin7 or ΔPIN7::PIN7–GFP/pin7 was indistinguishable. In contrast, 14-day-old ΔPIN7::PIN7–GFP/pin7 roots were significantly longer than control PIN7::PIN7–GFP/pin7 roots ( Fig. 1f,h ). Furthermore, truncation of the PIN7 promoter strongly interfered with the cytokinin sensitivity of root growth ( Fig. 1g,h ), root meristem size ( Fig. 1i ), lateral root initiation and development ( Fig. 1g,j ). Some phenotype features, such as primary root growth and its resistance to cytokinin, were comparable to the pin7 phenotype. However, reduced sensitivity of the root meristem as well as of the lateral root initiation to cytokinin were more pronounced in ΔPIN7::PIN7–GFP/pin7 seedlings. While we cannot exclude that these phenotypes are influenced by a change in the basal expression levels of PIN7 , on the basis of the altered cytokinin sensitivity of the transgenics, we suggest that regulation of PIN7 by cytokinins via PCRE7 is required for proper root growth and development. CRFs control PIN7 transcription To identify the upstream regulatory factors that control PIN7 transcription by direct interaction with PCRE7 , we employed an yeast one-hybrid (Y1H) assay. We screened the REGIA open reading frame (ORF) library that contains a set of ∼ 1,300 Arabidopsis transcription factors (TFs) and transcriptional regulators [22] . The Y1H screen with PCRE7 as bait ( Supplementary Fig. 3a ), identified CRF2, CRF3, and CRF6 that belong to the cytokinin-inducible subset of the APETALA2 (AP2)/ETHYLENE RESPONSIVE FACTOR family of TFs [21] ( Fig. 2a ). To confirm that the CRFs physically interact with PCRE7 , we analysed the CRF2::CRF2–GFP and 35S::CRF6–GFP transgenic plants through chromatin immunoprecipitation (ChIP) followed by quantitative PCR assays (ChIP–qPCR). Chromatin immunoprecipitated with anti-GFP antibodies was profoundly enriched in the PCRE7 region. No enrichment was detected when other distant sequences in the PIN7 ( PIN7 (-553-357)) promoter were tested ( Fig. 2c,d ; Supplementary Fig. 1c ). Hence, CRFs are directly associated with the PCRE7 . 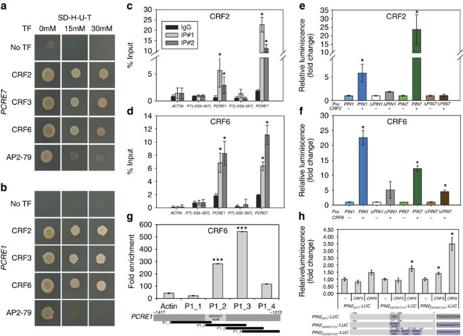Figure 2: Cytokinin response factors interact withPCREs. (a,b) CRF2, CRF3 and CRF6 interaction withPCRE7(a) andPCRE1(b) results in HIS3 reporter activation in an Y1H assay in contrast to AP2-79 that does not interact. Yeast cells were grown on SD-H-U-T minimal media without histidin (H), uracil (U) and tryptophan (T), supplemented with 3-amino-1,2,4-triazole (3AT). (c,d) Interaction of CRF2 (c) and CRF6 (d) withPCRE1andPCRE7detected by chromatin immunoprecipitation (ChIP). Chromatin immunoprecipitated with anti-GFP antibody is enriched in thePCRE1andPCRE7region. No enrichment was detected withPIN7(-553-357) andPIN1(-512-433) elements. (e,f) Significantly upregulated expression ofPIN1::LUCandPIN7::LUC, by co-expression withCRF2(e) andCRF6(f) in contrast to their truncated counterparts (ΔPIN1::LUC,ΔPIN7::LUC) inArabidopsismesophyll protoplasts, Student'st-test (*P<0.01,n=3). (g) ChIP of CRF6–GFP reveals a significantly higher enrichment for regions either containing (P1_2) or directly neighbouring (P1_3) the 5′-AGCAGAC-3′ motif when compared with more distant regions inPCRE1(P1_1 and P1_4) (***P<0.0001,n=3) (h). CRF6 increases expression ofPIN2promoter containing threeG2G5C7motifs inArabidopsisroot cell suspension protoplasts (*P<0.01,n=5) (h). Error bars represent s.e. (protoplast assay) and s.d. (ChIP). Experiments were repeated at least three times. Figure 2: Cytokinin response factors interact with PCREs . ( a , b ) CRF2, CRF3 and CRF6 interaction with PCRE7 ( a ) and PCRE1 ( b ) results in HIS3 reporter activation in an Y1H assay in contrast to AP2-79 that does not interact. Yeast cells were grown on SD-H-U-T minimal media without histidin (H), uracil (U) and tryptophan (T), supplemented with 3-amino-1,2,4-triazole (3AT). ( c , d ) Interaction of CRF2 ( c ) and CRF6 ( d ) with PCRE1 and PCRE7 detected by chromatin immunoprecipitation (ChIP). Chromatin immunoprecipitated with anti-GFP antibody is enriched in the PCRE1 and PCRE7 region. No enrichment was detected with PIN7 (-553-357) and PIN1 (-512-433) elements. ( e , f ) Significantly upregulated expression of PIN1::LUC and PIN7::LUC , by co-expression with CRF2 ( e ) and CRF6 ( f ) in contrast to their truncated counterparts ( ΔPIN1::LUC , ΔPIN7::LUC ) in Arabidopsis mesophyll protoplasts, Student's t -test (* P <0.01, n =3). ( g ) ChIP of CRF6–GFP reveals a significantly higher enrichment for regions either containing (P1_2) or directly neighbouring (P1_3) the 5′-AGCAGAC-3′ motif when compared with more distant regions in PCRE1 (P1_1 and P1_4) (*** P <0.0001, n =3) ( h ). CRF6 increases expression of PIN2 promoter containing three G2G5C7 motifs in Arabidopsis root cell suspension protoplasts (* P <0.01, n =5) ( h ). Error bars represent s.e. (protoplast assay) and s.d. (ChIP). Experiments were repeated at least three times. Full size image To gain insight into the role of the CRFs in the regulation of PIN transcription, we performed a transient expression assay in Arabidopsis protoplasts. The expression of the PIN7::LUCIFERASE ( LUC ) reporter was strongly activated when co-expressed with CRF2 and CRF6 ( Fig. 2e,f ), but not with CRF3 driven by constitutive 35S promoter ( Supplementary Fig. 3b ). Noteworthy, when co-expressed, CRF3 significantly attenuated the positive effect of CRF6 on PIN7::LUC expression ( Supplementary Fig. 3c ), indicating that individual CRFs might regulate PIN7 transcription differentially. No increase in the LUC reporter expression was detected when CRF2 was co-expressed with the truncated ΔPIN7::LUC construct ( Fig. 2e ). Co-expression with CRF6 stimulated ΔPIN7::LUC expression, but less when compared with the effect on the PIN7::LUC ( Fig. 2f ) thus further confirming the importance of the PCRE7 for CRF-dependent transcription. Collectively these data demonstrate that CRFs contribute to the transcriptional control of the PIN7 gene through physical interaction with a specific domain in its promoter. CRFs regulate transcription of PIN1 auxin efflux carrier Next we examined whether other PIN family members are transcriptionally controlled by CRFs similarly to PIN7 . Using promoter deletion analysis, we found that removal of the 200 bp between 1,417 and 1,212 bp upstream of the ATG codon resulted in cytokinin insensitivity of PIN1 transcription, hinting at the presence of the PCRE1 cis -regulatory element mediating cytokinin-induced transcriptional control in the PIN1 promoter ( Supplementary Figs 1b and 4a–e ). An Y1H assay confirmed an interaction of CRF2, CRF3 and CRF6 with this element ( Fig. 2b ; Supplementary Fig. 3a ). Accordingly, chromatin immunoprecipitated with anti-GFP antibodies from CRF2::CRF2–GFP and 35S::CRF6–GFP transgenic plants was profoundly enriched in the PCRE1 , while no enrichment was detected for distant sequence in the PIN1 promoter ( PIN1 (−512–433)) ( Fig. 2c,d ). The expression of PIN1::LUC , but not of ΔPIN1::LUC , was strongly activated when transiently co-expressed with CRF2 and CRF6 , in protoplasts ( Fig. 2e,f ). Similar to PIN7 , CRF3 did not significantly affect PIN1::LUC expression, but attenuated the CRF6 -stimulatory effect when co-expressed ( Supplementary Fig. 3d,e ). Altogether, these results indicate that PIN1 and PIN7 share common upstream regulatory components controlling their expression in response to cytokinin. PCRE1 and PCRE7 contain motifs recognized by CRFs Alignment of PCRE1 and PCRE7 elements with the Align programme (based on the ClustalW algorithm) [23] displayed a 54% sequence identity, suggesting that the cytokinin-dependent regulation of PIN1 and PIN7 might be governed by TFs recognizing common types of regulatory motifs. Previously, the GCC box (5′-AGCCGCC-3′) has been proposed as a binding motif recognized by ETHYLENE RESPONSE FACTOR1 (ERF1), a TF of the AP2/ERF family [21] , [24] , including CRF2, CRF3 and CRF4 (ref. 25 ). Scanning of PIN1 and PIN7 promoters revealed that neither PCRE1 nor PCRE7 contains a GCC box, and there is one GCC box located at (−483 bp) upstream of ATG in the PIN1 promoter ( Supplementary Fig. 1d ). However, no significant enrichment for the PIN1 fragment (-512-433) which contains this motif was detected using the ChIP–qPCR assay, indicating that CRF2 and CRF6 do not exhibit an increased affinity to this binding site ( Fig. 2c,d ). Noteworthy, several studies demonstrated that nucleotides G2 , G5 and C7 at conserved positions might be essential for the recognition of the GCC -derived motif by TFs of the AP2/ERF family [26] . We found that PCRE1 and PCRE7 contain 5′-AGCAGAC-3′ and 5′-AGAAGAC-3′ motifs, respectively, with critical nucleotides at conserved positions ( Fig. 2g ; Supplementary Fig. 1c,d ). To examine the relevance of these motifs for CRF binding, we tested whether CRF6 associates with them by ChIP–qPCR. Using specific primer combinations, we inspected enrichment for the short fragments spanning PCRE1 (ref. 27 ). Significantly increased enrichment detected for fragments either containing or directly neighbouring the 5′-AGCAGAC-3′ site when compared with more distant fragments in PCRE1 , strongly supports this motif as a CRFs’ recognition site ( Fig. 2g ). Additional thorough scanning for the presence of G2 , G5 and C7 motifs revealed one more motif in both PIN1 , as well as PIN7 promoters ( Supplementary Fig. 1c,d ). To further support our conclusion on the CRF-mediated regulation of PIN expression, we tested whether the PIN2 promoter, previously found to be cytokinin insensitive [28] might be activated by CRF after introducing the 5′-AGAAGAC-3′ motif. Detailed scanning of the PIN2 promoter sequence revealed that there are no 5′-AGCAGAC-3′ and 5′-AGAAGAC-3′ motifs present in the PIN2 promoter sequence within 2,500 bp upstream of the translation start and there is one 5′-GCCGTC-3 motif located at (−698 bp) upstream of the translational start. When the PIN2::LUC reporter was co-expressed with CRF6, a 1.47±0.38-fold increase of LUC activity (± indicates s.e., n =5) was detected, indicating modest CRF6 activity for the regulation of PIN2 promoter ( Fig. 2h ). Replacement of the 5′-GCCGTC-3′ motif in the PIN2 promoter by either one or three copies of the 5′-AGAAGAC-3′ motif resulted in a 1.75±0.17- and 3.48±1.02-fold increase of the LUC activity, respectively ( Fig. 2h ; ± indicates s.e., n =5). Hence, insertion of the 5′-AGAAGAC-3′ motif in triplicate into the PIN2 promoter significantly increased sensitivity to CRF6 ( Fig. 2h ), thus corroborating relevance of the motif identified in the PCRE7 element for CRF6-mediated expression. In line with previous observations, no dramatic effect on PIN2 , as well as on the PIN2 promoter containing PCRE7 motifs could be detected when co-expressed with CRF3 ( Fig. 2h ). Previously, type-B ARRs have been proposed to mediate cytokinin regulation of PIN1 and PIN7 expression through direct transcriptional control of the IAA3/SHY2 repressor of auxin signalling [10] . Three type-B ARRs (ARR10, ARR11 and ARR14) tested in an Y1H assay did not exhibit interaction with either PCRE1 or PCRE7 , which indicates that cytokinin transcriptional regulation of PIN1 and PIN7 might not occur by their direct binding to PCREs ( Supplementary Fig. 3f ). Altogether, these data suggest that CRF2 and CRF6 might recognize specific motifs within PCRE1 and PCRE7 with G2 , G5 and C7 at conserved positions to control PIN1 and PIN7 expression. Expression of PIN7 and PIN1 is altered in crf mutants The initial expression analysis revealed that the expression patterns of CRFs ,and PIN1 and PIN7 largely overlap in roots [29] ( Supplementary Fig. 5 compared with Fig. 1a and Supplementary Fig. 4a,c ), supporting their role as direct transcriptional regulators. To evaluate the impact of CRFs on PIN7 and PIN1 expression in planta , we examined lines with a modulated activity of CRFs ( Supplementary Fig. 6 ). Analyses of PIN7 expression using quantitative reverse transcription–PCR (qRT–PCR), as well as monitoring of PIN7::PIN7–GFP , PIN7::GUS , PIN7::GFP and PIN7::PIN7-GUS reporters revealed a significant increase of PIN7 expression in the root provasculature of RPS::CRF2 and 35S::CRF6 , but not of 35S::CRF3 lines ( Fig. 3a,b,e and Supplementary Fig. 7a–j ). This is largely in agreement with the results of a transient protoplast assay ( Fig. 2e,f compared with Fig. 3a,b,e ). Lack of the PCRE7 in the ΔPIN7::PIN7–GFP line interfered with the stimulatory effect of CRF2 on PIN7–GFP expression, regardless of cytokinin levels ( Fig. 3c,d ). Analysis of PIN7 expression using PIN7::PIN7–GFP and PIN7::GUS reporters, as well as qRT–PCR in mutants lacking either of the CRFs revealed attenuated PIN7 expression in crf3 , as well as crf2crf3crf6 roots and enhanced PIN7 expression in crf6 roots ( Supplementary Fig. 7k–s ). 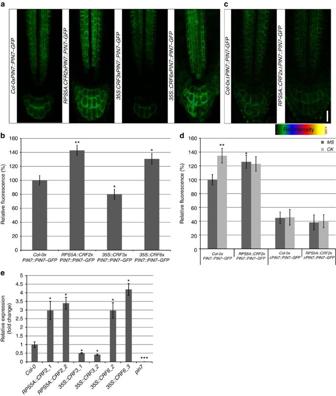Figure 3: Expression ofPINgenes is altered inCRF-overexpressing lines. (a,b)PIN7::PIN7–GFPexpression is upregulated in the provasculature ofCRF2andCRF6, but downregulated inCRF3-overexpressing lines. (c,d)ΔPIN7::PIN7–GFPis not upregulated in theCRF2-overexpressing line in either absence or presence of cytokinin (5 μM N6-benzyladenine for 5 h). The membrane PIN7–GFP signal was quantified in the pericycle (b,d). Student'st-test (*P<0.05, **P<0.01;n=15–20). (e)PIN7expression in lines overexpressing CRFs monitored by qRT–PCR, no expression detected inpin7mutant (*P<0.05; ***P<0.0001,n=3). Error bars represent s.e. Seven-day-old seedlings were analysed. Scale bar, 20 μm. Three independent experiments were performed giving the same statistically significant results. Figure 3: Expression of PIN genes is altered in CRF -overexpressing lines. ( a , b ) PIN7::PIN7–GFP expression is upregulated in the provasculature of CRF2 and CRF6 , but downregulated in CRF3 -overexpressing lines. ( c , d ) ΔPIN7::PIN7–GFP is not upregulated in the CRF2 -overexpressing line in either absence or presence of cytokinin (5 μM N6-benzyladenine for 5 h). The membrane PIN7–GFP signal was quantified in the pericycle ( b , d ). Student's t -test (* P <0.05, ** P <0.01; n =15–20). ( e ) PIN7 expression in lines overexpressing CRFs monitored by qRT–PCR, no expression detected in pin7 mutant (* P <0.05; *** P <0.0001, n =3). Error bars represent s.e. Seven-day-old seedlings were analysed. Scale bar, 20 μm. Three independent experiments were performed giving the same statistically significant results. Full size image Similar to PIN7 , PIN1 expression was significantly upregulated in roots overexpressing CRF2 as detected by using PIN1::PIN1–GFP and PIN1::GFP reporters, as well as by qRT–PCR. Deletion of the PCRE1 in the ΔPIN1::PIN1–GFP line interfered with the stimulatory effect of CRF2 on PIN1 expression in agreement with the proposed role of the PCRE1 in CRF-dependent transcriptional control ( Supplementary Fig. 8a–d ). Inspection of crf loss-of-function mutants further confirmed the role of CRFs in the regulation of PIN1 expression in planta . PIN1 expression was significantly reduced in crf2 , crf3 , crf3crf6 and crf2crf3crf6 loss-of-function mutants ( Supplementary Fig. 8e–g ), thus resembling the PIN7 expression pattern in these mutant backgrounds. Altogether, the expression analysis data support a role of the CRFs in balancing the PIN7 and PIN1 transcription. Nevertheless, inconsistency in PIN7 and PIN1 expression patterns observed in lines with modulated CRF expression, such as downregulation of both PIN1 and PIN7 in crf3 , and upregulation in crf6 , might reflect the presence of intricate in planta regulatory mechanisms, for example, the existence of a transcriptional complex in which additional components could function as modifiers. This is strongly supported by recent observations that individual CRFs might interact with other family members, as well as with type-B ARRs [30] . Collectively, our data demonstrate that CRFs contribute to balancing PIN7 and PIN1 expression and that CRF homologues might have specific functions in the control of PIN expression. CRFs mutants display an auxin transport-defective phenotype To examine a role of CRFs as direct upstream regulators of PIN transcription, we analysed in detail the phenotype of plants with modulated CRF expression. Altered expression of PINs in crf loss-of-function mutants might result in an abnormal auxin distribution and, consequently, in developmental and patterning defects as previously demonstrated for auxin distribution mutants [1] , [31] . Indeed, auxin measurements in root tips of crf3crf6 mutants revealed an increase in auxin levels ( Fig. 4a ). Similarly, the auxin accumulation at root tips of a mutant lacking PIN4 auxin efflux carrier activity has been previously observed [31] . 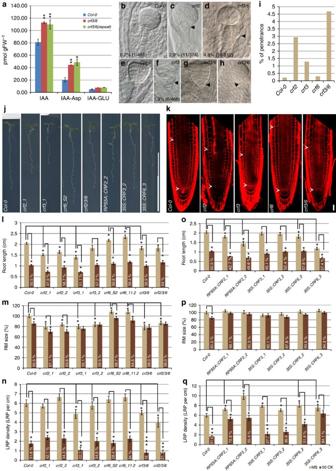Figure 4:crfmutants exhibit defective embryogenesis and root development. (a) Auxin accumulation in the root tip ofcrf3crf6mutants. (b–i) Abnormal divisions of upper suspensor cells, embryo proper and occasionally double embryos were observed in embryos ofcrf2(c),crf3(f) andcrf3crf6(d,g,h) loss-of-function mutants when compared with controls (b,e,i). (j–n) Lack ofcrf2,crf3,crf6, as well ascrf3crf6andcrf2crf3crf6function affects root length (j,l), root meristem size (k,m), and lateral root primordia density (n) and their response to cytokinin. (o–q) Constitutive expression ofCRF2,CRF3andCRF6affects root growth (o), root meristem size (p), and lateral root initiation density (q) and their response to cytokinin. Seedlings were grown for 7 days on control MS medium with or without 0.05 μM of the cytokinin (CK) N6-benzyladenine (l–q). Student'st-test (*P<0.05; **P<0.01; ***P<0.001;n=10–15). Arrows indicate the distance between the quiescent centre (QC) and the cortex transition zone (k). Error bars represent s.e. Scale bars, (b–h) 10 μm (j) 2 cm, (k) 20 μm. The graphs show the results of one biological repeat, representative for two additional independent experiments. Figure 4: crf mutants exhibit defective embryogenesis and root development. ( a ) Auxin accumulation in the root tip of crf3crf6 mutants. ( b – i ) Abnormal divisions of upper suspensor cells, embryo proper and occasionally double embryos were observed in embryos of crf2 ( c ), crf3 ( f ) and crf3crf6 ( d , g , h ) loss-of-function mutants when compared with controls ( b , e , i ). ( j – n ) Lack of crf2 , crf3 , crf6 , as well as crf3crf6 and crf2crf3crf6 function affects root length ( j , l ), root meristem size ( k , m ), and lateral root primordia density ( n ) and their response to cytokinin. ( o – q ) Constitutive expression of CRF2 , CRF3 and CRF6 affects root growth ( o ), root meristem size ( p ), and lateral root initiation density ( q ) and their response to cytokinin. Seedlings were grown for 7 days on control MS medium with or without 0.05 μM of the cytokinin (CK) N6-benzyladenine ( l – q ). Student's t -test (* P <0.05; ** P <0.01; *** P <0.001; n =10–15). Arrows indicate the distance between the quiescent centre (QC) and the cortex transition zone ( k ). Error bars represent s.e. Scale bars, ( b – h ) 10 μm ( j ) 2 cm, ( k ) 20 μm. The graphs show the results of one biological repeat, representative for two additional independent experiments. Full size image By closer examination of plants lacking CRF activity, developmental abnormalities were found reminiscent of those caused by impaired auxin transport. A significantly enhanced number of embryonic defects, such as abnormal divisions of upper suspensor cells and in the embryo proper, and occasionally the appearance of double embryos, was observed in embryos of crf2 , crf3 and crf3crf6 loss-of-function mutants when compared with control lines ( Fig. 4b–i ), thus phenocopying the pin1 , pin7 and multiple pin embryo defects [1] . Accordingly, CRF2 , CRF3 and CRF6 expression was detected in early embryos ( Supplementary Fig. 5 ). Lack of functional CRF2, CRF3, both CRF3 and CRF6 or CRF2, CRF3, CRF6 correlated with reductions in root length, root meristem size and lateral root initiation ( Fig. 4j–n ), which are developmental aberrations typically associated with defective auxin transport [3] , [32] , [33] . On the contrary, crf6 loss-of-function mutants, in which PIN7 expression was enhanced, exhibited longer roots and a larger root meristem ( Fig. 4j–n ). Altogether, modulation of CRF activity alters auxin accumulation in the root tips, and leads to developmental defects in many aspects, mimicking phenotypes of auxin distribution mutants [1] , [31] , [32] . CRFs fine-tune root system response to cytokinin and auxin Typically, an increase in cytokinin activity alters root growth and development: cytokinins restrict root elongation growth, cause shortening of the root meristem size, and compromise the initiation and development of the lateral roots [4] , [5] , [10] , [11] , [34] , [35] . While cytokinin inhibitory effects of root elongation involves ethylene [11] , [34] , reduction of the root meristem size, as well as lateral root initiation by cytokinin occurs largely in an ethylene independent manner [5] , [11] . To examine the possible role of CRFs in cytokinin-mediated root system establishment, lines with modulated CRF activity were exposed to increased cytokinin concentrations. We found that neither gain nor loss of CRF activity dramatically changed root growth response to cytokinin ( Fig. 4l,o ). The root meristem cytokinin response was unaffected in crf2 and crf6 mutants and reduced in crf3 and crf3crf6 , as well as crf2crf3crf6 mutants ( Fig. 4m ). Constitutive expression of CRF2 , CRF3 and CRF6 reduced root meristem response to cytokinin ( Fig. 4p ). Noteworthy, most pronounced changes were observed in cytokinin effect on lateral root initiation and development. The significant increase in cytokinin inhibitory effects on both lateral root initiation and development was detected in crf3, crf3crf6 and crf2crf3crf6 mutants ( Fig. 4n ; Supplementary Fig. 9a–e ), whereas CRF2 and CRF6 overexpression attenuated cytokinin effects ( Fig. 4q ; Supplementary Fig. 9f,g ). In contrast to cytokinin, root system response to auxin was reduced in crf3 , crf3crf6 and crf2crf3crf6 mutants, which was manifested by an attenuated stimulatory effect of auxin on lateral root initiation ( Supplementary Fig. 10a–e ). Constitutive expression of CRF2 led to significantly enhanced response to auxin, whereas no dramatic changes in lateral root initiation after auxin treatment in either the CRF3 or CRF6 overexpressor line when compared with the wild-type control were detected ( Supplementary Fig. 10f–h ). Hence, perturbations in CRF expression affect root response to cytokinin and auxin, and indicate that CRFs by control of auxin transport might fine-tune cytokinin- and auxin-mediated root growth and development. Auxin gradients represent universal mechanisms to control plant organogenesis. Modulation of the activity of the transport machinery that regulates auxin distribution directly impacts on organ formation and patterning and, thus, accounts for a developmentally efficient tool to flexibly adapt plant architecture depending on the changing environmental conditions. Recently, evidence accumulates that exogenous factors, such as light or gravity, through their endogenous counterpart, that is, plant hormones including ethylene, gibberellin, jasmonate and cytokinin, modulate the activity of the polar auxin transport machinery to direct plant growth and development [10] , [11] , [19] , [36] , [37] , [38] , [39] . However, the molecular basis of these regulations are scarcely understood so far. Here we demonstrate that the expression of auxin efflux transporters can be effectively uncoupled from cytokinin control through deletion of the PCRE cis -regulatory element in the promoter of the PIN auxin efflux carrier gene. Moreover, we found that the activity of the ΔPIN7 promoter lacking PCRE7 was significantly reduced in the root provasculature and in columella cells when compared with the full PIN7 promoter, indicating the importance of this promoter element for the regulation of basal PIN7 expression and it suggests that cytokinin might participate in the establishment and maintenance of the proper expression level of PIN7 through this regulatory element. Truncation of the PIN7 promoter causes loss of cytokinin-dependent PIN7 transcription and impacts on cytokinin-mediated root growth and branching. While it is difficult to conclusively attribute these phenotypes directly to the loss of cytokinin sensitivity as opposed to a change in basal expression levels, the altered cytokinin responsiveness of the transgenic plants suggests, that tightly controlled PIN-dependent auxin transport may be significant in the establishment of the root system architecture. Attempts to reveal components of the upstream regulatory pathway acting at the PCRE led to the identification of CRFs as direct transcriptional regulators. Originally, CRFs have been found as a subgroup of the AP2 family of TFs, which are rapidly induced by cytokinin, and they have been proposed to mediate the transcriptional response to cytokinin [21] . However, the CRFs’ downstream targets and pathways remained unknown so far. Here we show that through interaction with the cis -regulatory PCRE , presumably through recognition of the 5′-AGCAGAC-3′-like motif, CRFs control expression of PIN1 and PIN7 . Interestingly, although PIN7 and PIN1 share common molecular components mediating transcriptional regulation by cytokinin, the expression of PIN7 is upregulated, whereas expression of PIN1 is downregulated in response to exogenous cytokinin. The finding that PIN transcription is differentially controlled by individual CRFs, for example, CRF3 counteracts both CRF2- as well as CRF6-stimulatory effects, indicates that the final output might depend on the balance between individual CRFs and their mutual interactions [30] in certain tissues. It is also possible that the transcriptional activity of individual CRFs can be attenuated by additional molecular modifiers. Modulation of the CRF activity results in significant changes of the PIN1 and PIN7 expression patterns and in phenotype aberrations reminiscent of mutants with defective auxin transport [1] , [31] , [32] . This, together with a significant overlap in the expression of PIN and CRF genes during embryogenesis, in the root meristems and LRP, strongly supports a role of CRFs in the regulation of PIN expression. Accordingly, the expression of several CRFs in vascular tissue has been correlated with alterations of the vascular patterning in CRF loss-of-function mutants [40] , similarly to those observed in auxin transport mutants [41] . In this light, the identification of the PIN genes as direct targets of CRFs reveals a missing direct regulatory link between the cytokinin signalling and the auxin transport machinery. Moreover, CRF2 ( TARGET OF MONOPTEROS ( TMO3 )) as a direct transcriptional target of the AUXIN RESPONSE FACTOR5 / MONOPTEROS [42] might account for an important convergence point to the previously characterized AHK3-ARR , ARR12-IAA3 / SHY2 regulatory chain [10] and balance both auxin and cytokinin input to control auxin transport. Furthermore, the recent observation that CRF6 is induced by numerous stresses [29] hints at a role of CRFs as factors modulating auxin transport in response to environmental signals. Plant material and growth conditions The transgenic Arabidopsis thaliana (L.) Heynh. lines have been described elsewhere: PIN1::PIN1–GFP [3] , pin7-2 (ref. 3 ), PIN7::PIN7–GFP [32] , PIN7::GUS [1] , RPS5A::CRF2 (ref. 42 ), 35S::EGFP-CRF6 (ref. 43 ). The previously characterized CRF knockout mutants [21] were obtained from various T-DNA insertion mutant seed collections: crf2-1, crf2-2 , crf3-1 and crf3-2 from the Salk Institute Genomic Analysis Laboratory (SAIL, former GARLIC) T-DNA insertion lines from the Torrey Mesa Research Institute [44] and crf6-S2 and crf6-11.2 from GABI-Kat [45] . The crf3crf6 double and crf2crf3crf6 triple mutants were generated from crf3-1 , crf6-S2 and crf2-2 , and crf3-1 and crf6-S2 respectively. Primers and T-DNA accession numbers are listed in Supplementary Table 1 . Seeds of Arabidopsis (accession Columbia-0) were plated and grown on square plates with solid half-strength Murashige and Skoog (MS) medium supplemented with 0.5 g l −1 MES, 10 g l −1 Suc and 0.8% agar. The plates were incubated at 4 °C for 48 h to synchronize seed germination and then grown vertically in growth chambers under a 16:8 h day/night cycle photoperiod at 18 °C. Cytokinin treatments were performed with the N6-benzyladenine cytokinin derivative, concentrations were adapted to the experimental setups. Typically, to examine root growth response to cytokinin, low 0.25, 0.5 and 0.1 μM cytokinin concentrations were applied. The cytokinin impact on PIN expression was examined 8 h after treatment with cytokinin, therefore higher concentrations of 2 and 5 μM were applied. Cloning and generation of transgenic lines For promoter analysis of PIN1 and PIN7 , particular promoter fragments were amplified by PCR and cloned into the pGEM-T vector. The used primers contained unique restriction sites: PstI-sense and BamHI-antisense for PIN1, and SalI-sense and BamHI-antisense for PIN7 , allowing digestion and subsequent cloning into the pGREEN binary vector. The resulting constructs contained transcriptional fusions between the PIN1 or PIN7 promoter variants and the enhanced GFP with a nuclear localization signal (NLS). Primers used for cloning are listed in Supplementary Table 2 . The translational fusion ΔPIN1::PIN1–GFP was obtained by modifying PIN1::PIN1–GFP (in pBINPLUS vector backbone [3] ) as follows: the PIN1 promoter sequence from −258 to −2,320 relative to the initiating ATG was removed by XbaI digestion and replaced by the PIN1 promoter sequence spanning the −258 to −1,212 region. ΔPIN7::PIN7–GFP was derived from PIN7::PIN7–GFP in pBINPLUS [1] by removal of the EcoRI fragment. The truncated promoter construct contained 1,141 bp upstream of the translational start site. Expression plasmids were generated by standard molecular biology protocols and Gateway technology (Invitrogen). ORFs were amplified from a complementary DNA (cDNA) template with Pfu DNA Polymerase (Promega, Madison, WI, USA) and fused to the Gateway attB sites by PCR. pDONR221 and p4-p1r were used as ENTRY vectors. The structure and sequence of all destination vectors were as described [46] , [47] and are available online at http://www.psb.ugent.be/gateway/ or otherwise referenced. 35S::CRF3 and 35S::CRF6 were obtained by cloning the ORFs of CRF3 and of CRF6 into destination vectors pK7WG2.0 and pK7WG2D , respectively. Overexpression of these lines was confirmed by qPCR, primers are included in Supplementary Table 2 . The CRF3 and CRF6 (2 kb) promoters were cloned in pMK7S*NFm14GW , generating the ProCRF3:NLS–GFP–GUS and ProCRF6:NLS–GFP–GUS constructs (transcriptional fusions between the promoters and the gene encoding the EGFP-GUS fusion protein), respectively. The CRF2::CRF2–GFP fusion, used for the ChIP experiments, was generated by cloning a DNA fragment consisting of the 2-kb CRF2 proximal promoter and the CRF2 coding sequence in frame to 3 × GFP in the PgreenIIK vector. All transgenic plants were generated by the floral dip method [48] . At least two independent transgenic lines were examined for expression pattern. Quantitative RT–PCR RNA was extracted with the RNeasy kit (Qiagen) from excised root tips of 7-day-old root sample. A DNase treatment with the RNase-free DNase Set (Qiagen) was carried out for 15 min at 25 °C. Poly(dT) cDNA was prepared from 1 μg of total RNA with the iScript cDNA Synthesis Kit (Biorad) and analysed on a LightCycler 480 (Roche Diagnostics) with the SYBR Green I Master kit (Roche Diagnostics) according to the manufacturer’s instructions. Targets were quantified with specific primer pairs designed with the Beacon Designer 4.0 (Premier Biosoft International, Palo Alto, CA, USA). All PCRs were performed in triplicate. Expression levels were first normalized to ACTIN2 expression levels and then to the respective expression levels in the wild type. The primers used to quantify gene expression levels are listed in Supplementary Table 2 . Phenotypic analysis For root length analysis, seedlings were photographed and root lengths were measured with ImageJ ( http://rsb.info.nih.gov/ij ). To examine root growth kinetics, seedling growth was recorded daily during 14 days with an EOS035 Canon Rebel Xti camera. Long-term root growth observations for 28 days were performed on Petri dishes of 245 per 245 mm size. About 10–15 seedlings were processed, and 3 independent experiments were performed. To determine root meristem size, 7-day-old seedlings ( n =10–15) were stained with propidium iodide (1 μl ml −1 ) and microscopy was performed using Zeiss LSM 510 confocal microscope. The distances between the quiescent centre and the first elongating cell were measured with ImageJ. To score LRP density, 7-day-old seedlings ( n =10–20) were first processed by clearing [49] . In brief, seedlings were incubated in a solution containing 4% HCl and 20% methanol for 15 min at 57 °C, followed by 15 min incubation in 7% NaOH/60% ethanol at room temperature. Next, seedlings were rehydrated by successive incubations in 40, 20 and 10% ethanol for 5 min, followed by incubation (15 min up to 2 h) in a solution containing 25% glycerol and 5% ethanol. Finally, seedlings were mounted in 50% glycerol and root lengths were measured on scanned slides with ImageJ. Scoring of LRP was performed by using a DIC Olympus BX51 microscope. Histochemical and histological analysis To detect β-Glucuronidase (GUS) activity, 5-day-old seedlings were incubated in reaction buffer containing 0.1 M sodium phosphate buffer (pH 7), 1 mM ferricyanide, 1 mM ferrocyanide, 0.1% Triton X-100 and 1 mg ml −1 X-Gluc for 1 up to 24 h in dark at 37 °C. Afterwards, chlorophyll was removed by destaining in 70% ethanol and seedlings were cleared [49] as described above. GUS expression was monitored by differential interference contrast microscopy (Olympus BX51). Immunodetection of PIN1 expression in roots (5-day-old seedlings) and GFP reporter expression in CRF2::GFP transgenic embryos (harvested from siliques of ∼ 4-week-old plants) were performed using an automated system (Intavis in situ pro) according to published protocol [50] . Roots and embryos were fixed in either 4% paraformaldehyde or 4% paraformaldehyde and 0.1% Triton, respectively, for 1 h in vacuum at room temperature. Afterwards, seedlings were first incubated for 30–45 min in PBS (2.7 mM KCl,137 mM NaCl, 4.3 mM Na 2 HPO 4 2H 2 O and 1.47 mM KH 2 PO 4 , pH 7,4) containing 2% Driselase at 37 °C in a humid chamber, and then in PBS supplemented with 3% NP40 and 20% DMSO for 1 h at room temperature. After blocking with 3% BSA in PBS (3 h at 37 °C), samples were incubated with primary antibody (affinity-purified rabbit anti-yellow fluorescent protein polyclonal serum [42] and rabbit anti-PIN1 (ref. 51 ) polyclonal antibody diluted in blocking solution 1:600 and 1:1,000, respectively) for 2 h at 37 °C. Secondary antibody incubation was carried on for 2 h at 37 °C. Anti-rabbit-Alexa 488 (Sigma A-11034) and CY3-conjugated anti-rabbit antibody (Sigma, C2306) were diluted 1:600 in blocking solution. Control staining was done with propidium iodide diluted 1:1,000 in water. Samples were mounted in solution containing 25 mg ml −1 DABCO (Sigma) in 90% glycerol, 10% PBS, pH 8.5. Expression was monitored using a confocal laser scanning microscope (LSM 510, Zeiss). Images were analysed by using ImageJ software. Confocal imaging and image analysis Zeiss LSM 510, Zeiss LSM 710 or Olympus FV10 ASW confocal scanning microscopes using either × 20 or × 60 (water immersion) objectives were employed to monitor expression of fluorescent reporters. GFP and propidium iodide signals were detected either at 488 nm excitation/507 nm emission or 536 nm excitation/617 nm emission wavelength, respectively. For real-time analysis of PIN7–GFP expression in LRP, 6-day-old seedlings were placed on chambered cover glass (Nunc Lab-Tek) and covered with 0.2-mm-thin square blocks of solid 0.5 × MS media with or without cytokinin. LRPs were scanned in 30-min time intervals for 16 h by the FV10 ASW confocal microscope (Olympus). To evaluate relative PIN7–GFP expression levels, a minimum of 10 LRPs in stage-I positioned in the plane with two xylem strands were selected, and the PIN–GFP membrane signals at two anticlinal plasma membranes per LRP were measured. Quantification of PIN–GFP or immunodetected PIN expression in root meristems was performed by measurement of membrane signal in either pericycle or endodermal cells ( n =10 roots, five cells per root) using ImageJ. About 10–15 seedlings were analysed, the statistical significance was evaluated by Student’s t -test. Auxin accumulation in root tips of crf3crf6 double mutants Root tips (2-mm segments, about 100 mg) of 6-day-old A. thaliana (L.) Heynh. seedlings grown on vertical plates were separated and collected in 300 μl Bieleskis solution and homogenized. After overnight extraction at −20 °C, the tissues were separated by centrifugation (15,000 g ) and extracts were evaporated to dryness. Quantification of auxin and auxin metabolites was performed by HPLC-MS/MS according to ref. 52 , in short: dried samples were dissolved in 50 μl 10% (v/v) acetonitrile in water and centrifuged (15,000 g , 10 min, 4 °C). An aliquot (10 μl) of each supernatant was separately applied to HPLC (Ultimate 3000, Dionex) coupled to a hybrid triple quadrupole/linear ion trap mass spectrometer (3200 Q TRAP, Applied Biosystems). Calibration was performed using a multilevel calibration graph with (2H)-labelled internal standards. Results represent the mean of three independent repeats for each sample. Y1H screen The yeast strain YM4271 and destination vectors pDEST-MW1 and pDEST- MW2 have been previously described [53] . Yeast reporter strains were designed as described [53] . For the Y1H cDNA library screen, the 200-bp promoter fragments PCRE1 and PCRE7 were cloned into the destination vectors pDEST-MW1 and pDEST- MW2 , respectively, by Gateway cloning (for primers sequences see Supplementary Table 2 ). The DNA baits were integrated into yeast using the high efficiency transformation protocol according to the Yeast Protocol Handbook (Clontech) except that 1 μg of linearized plasmid DNA was added to the competent yeast, the heat shock period at 42 °C was extended to 20 min and the cells were resuspended in 150 μl TE buffer. The cDNA Y1H library screen was performed with a REGIA and REGULATORS (RR) collection, previously described [22] . For the transformation of one TF, 20 μl of competent yeast, 2 μl of carrier DNA, 100 ng plasmid (TF) DNA and 100 μl of TE/LiAC/PEG were used. Yeast cells were resuspended in 20 μl TE buffer and spotted on SD-His-Ura-Trp medium. After 3 days of growing, replica plates were made with 0, 15 and 30 mM 3-aminotriazole and positive clones were selected after 6 to 8 days of incubation at 30 °C. Transient expression in Arabidopsis mesophyll protoplasts Mesophyll protoplasts were isolated from rosette leaves of 4-week-old Arabidopsis plants grown in soil under controlled environmental conditions in a 16:8 h light/dark cycle or under continuous light at 21 °C. Protoplasts were isolated and transient expression assays were carried out as described [54] with modifications [55] . Protoplasts were co-transfected with 20 μg of a reporter plasmid that contained fLUC , a reporter gene driven by the corresponding promoter, 2 μg of normalization plasmid expressing the Renilla LUC ( rLUC ) under the control of the 35S promoter and 20 μg of the effector construct. For the reporter constructs, the pEN-L4-Pro-R1 vector (with Pro representing PIN1:LUC , ΔPIN1::LUC , PIN7::LUC , and ΔPIN7::LUC ) was recombined together with pEN-L1-fLUC-L2 by Multisite Gateway LR cloning with pm42GW736 . For the effector constructs, the pEN-L1-ORF-R2 plasmids (with the ORF of CRF2 , CRF3 or CRF6 ) were used to introduce the ORFs by Gateway LR cloning into p2GW7 for overexpression. The total amount of DNA was equalized in each experiment with the p2GW7-GUS mock effector plasmid. After transfection, protoplasts were incubated overnight and then lyzed; fLUC and rLUC activities were determined with the Dual-Luciferase reporter assay system (Promega). Variations in transfection efficiency and technical errors were corrected by normalization of fLUC by the rLUC activities. The mean value was calculated from three measurements and each experiment was repeated at least three times. Transient expression in root syspension culture protoplasts The LUC assays were performed from 3-days-old Arabidopsis root suspension culture by PEG mediated transformation. Protoplasts were isolated in enzyme solution (1% cellulose;Yakult, 0.2% Macerozyme;Yakult in B5-0.34M glucose-mannitol solution; 2.2 g MS with vitamins, 15.25 g glucose, 15.25 g mannitol, H2O to 500 ml pH to 5.5 with KOH) with slight shaking for 3–4 h, centrifuged at 800 g for 5 min. The pellet was washed with B5-0.34M glucose-mannitol solution and resuspended in B5-0.34M glucose-mannitol solution to a final concentration of 2 × 10 5 per 50 μl. 2 μg of reporter and effector plasmid DNAs were gently mixed together with 50 μl of protoplast suspension and 60 μl of PEG solution (0.1 M Ca(NO3)2, 0.45 M Mannitol, 25% PEG 6000) and incubated in the dark for 10 min. Then 140 μl of 0.275 M Ca(NO3)2 solution was added to wash off PEG, centrifuged at 800 g for 5 min and supernatant was removed. The protoplast pellet was resuspended in 200 μl of B5-0.34M glucose-mannitol solution and incubated for 16 h in the dark at room temperature. The LUC assays were performed using a Dual-Luciferase Reporter Assay System as described for mesophyll protoplasts above. For cloning of the PIN2wt:LUC construct, 1.5 kb fragment of the PIN2 promoter upstream from the translational start was PCR amplified from the genomic DNA using SalI-Fw and NcoI-Rv primers and the PCR product was subsequently cloned as SalI+NcoI fragment into the pGreen008-II-Luc vector [56] in frame with the coding sequence of the LUC gene. For introducing PCRE7 motives, mutagenesis by PCR-driven overlap extension technique was used as described previously in ref. 57 . Briefly, intermediate primers containing PCRE7 motives were designed with complementary ends and PCRs were performed using following primer combinations (listed in Supplementary Table 1 ): For introducing PCRE7-1 motif, SalI-Fw primer in combination with PCRE7-1-Rv and NcoI-Rv primer in combination with PCRE7-1 -Fw were used, and PIN2wt promoter DNA was used as template. The two PCRs products were purified and combined in equal concentrations and were subsequently used as template in the extension PCR round to get a full length PIN2 promoter with PCRE7-1 motif. Similarly for introducing PCRE7-3, SalI-Fw primer in combination with PCRE7-3-Rv and NcoI-Rv primer in combination with PCRE7-3-Fw were used, in this case and PIN2 promoter with PCRE7-1 motif was used as template. The two PCRs products were purified and combined in equal concentrations and were subsequently used as template in the extension PCR round to get a full length PIN2 promoter with PCRE7-3 motif. The PCR products were subsequently cloned into as SalI+NcoI fragment into the pGreen008-II-Luc vector. ChIP assay ChIP experiments were done as described [58] with minor modifications. One gram of tissue from 8-day-old plants was harvested and immersed in 1% formaldehyde under vacuum for 10 min. Glycine was added to a final concentration of 0.125 M and incubation was continued for 5 min. After washing, the nuclei were isolated and cross-linked DNA/protein complexes were fragmented by sonication with a Bioruptor sonicator (Diagenode), resulting in fragments of ∼ 500 bp. After centrifugation (at 500 g ), the supernatant was precleared with 80 μl of sheared salmon sperm DNA and protein A agarose (Millipore), of which 10 μl was used as input and the remainder was divided into three samples. To two samples (IP1 and IP2), 25 μl GFP–Trap_A coupled to agarose beads (Chromotec, gta-20) was added, whereas to the third sample, which served as IgG control, an equal volume of nonspecific control serum was added, consisting of sonicated salmon sperm DNA, BSA and protein A (salmon sperm DNA/protein A agarose-50% slurry). The samples were incubated overnight and immunoprecipitates were subsequently eluted from the beads. All centrifugation steps with bead-containing samples were done at 500 g . Proteins were de-cross-linked and DNA was purified by phenol/chloroform/isoamyl alcohol extraction and ethanol precipitation. Pellets were resuspended in MiliQ water. The concentration of ChIP DNA was measured with the Quant-iT double-stranded DNA HS assay kit (Invitrogen). The SYBR Green I Master kit was used for all qPCRs. ACTIN2 and promoter regions of PIN1 (433–512 bp upstream of the start codon) and PIN7 (357–553 upstream of the ATG) were utilized as negative controls. All primer sequences, including those for PCRE1 and PCRE7 , as well as primers used for identification of CRF motif are listed in Supplementary Table 2 . To analyse the ChIP enrichment from qPCR data, the Percent Input Method and Fold Enrichment Method were used. Each ChIP DNA fractions’ Ct value was normalized to the Input DNA fraction Ct value for the same qPCR Assay (ΔCt). ΔCt [normalized ChIP]=(Ct [ChIP]–(Ct [Input]–Log2 (Input Dilution Factor))). In which Input Dilution Factor (Fd)=1/100 (fraction of the input chromatin saved). The average of normalized ChIP Ct values for replicate samples was calculated. Percent Input was then calculated as: %input=2 (−ΔCt (normalized ChIP)) . The normalized ChIP fraction Ct value was adjusted for the normalized background (IgG) fraction Ct value (first ΔΔCt). ΔΔCt (ChIP/IgG)=ΔCt (normalized ChIP)–ΔCt (normalized IgG). IP Fold Enrichment above the sample specific background was calculated as linear conversion of the first ΔΔCt: Fold Enrichment=2 (−ΔΔCt (ChIP/IgG)) . S.d. was calculated for IP1 and IP2 as ln(2) × dSD × FC and for IgG as ln(2) × dSD, with FC the fold change. ChIP data were obtained from single experiments, but similar data were acquired from three independent experiments. How to cite this article: Šimášková, M. et al . Cytokinin response factors regulate PIN-FORMED auxin transporters. Nat. Commun. 6:8717 doi: 10.1038/ncomms9717 (2015).